Rad23 escapes degradation because it lacks a proteasome initiation region Rad23 is an adaptor protein that binds to both ubiquitinated substrates and to the proteasome. Despite its association with the proteasome, Rad23 escapes degradation. Here we show that Rad23 remains stable because it lacks an effective initiation region at which the proteasome can engage the protein and unfold it. Rad23 contains several internal, unstructured loops, but these are too short to act as initiation regions. Experiments with model proteins show that internal loops must be surprisingly long to engage the proteasome and support degradation. These length requirements are not specific to Rad23 and reflect a general property of the proteasome. Rad23 functions in both DNA repair and the ubiquitin–proteasome system [1] , [2] . After DNA is damaged by radiation, a complex of Rad23 and Rad4 binds to the DNA region containing the lesion and, together with a second complex, causes the excision of the damaged nucleotides [1] . In the ubiquitin–proteasome system, Rad23 binds both the proteasome and ubiquitinated proteins and is thought to function as an adaptor protein that delivers substrates to the proteasome for degradation [1] , [2] , [3] , [4] , [5] , [6] . Indeed, deletion of Rad23 together with the proteasome subunit Rpn10 leads to an accumulation of ubiquitinated proteins and overexpression of Rad23 inhibits degradation of proteins [5] , [6] , [7] , [8] , [9] , [10] , [11] , [12] . Rad23 in yeast is a 42 kDa protein and includes four domains: an amino (N)-terminal ubiquitin-like (UbL) domain, two ubiquitin-associated (UBA) domains, and a Rad4-binding domain (RBD) [1] (see schematic drawing in Fig. 1a ). These four domains have well-defined structures but are connected by flexible linker regions ranging in length from 45 to 82 amino acids [13] . The RBD links Rad23 to nucleotide excision repair [14] . The UbL domain allows Rad23 to bind to the proteasome [3] , [14] , where it is recognized by the Rpn1 (refs 15 , 16 ) and Rpn13 (ref. 17 ) subunits, and by human, but not yeast, Rpn10 (ref. 18 ). The UBA domains bind to ubiquitin, UbL domains, or ubiquitinated proteins [10] , [19] , [20] , [21] , [22] . Rad23's binding to both the proteasome and ubiquitinated proteins allows it to function as an adaptor protein that delivers substrates to the proteasome for degradation [2] , [4] , [5] , [6] . Rad23 belongs to a larger group of targeting adaptors, which includes the proteins Dsk2 and Ddi1 in yeast and a larger number of proteins in mammalian cells [2] , [19] , [21] , [23] , [24] . These adaptors are defined by the presence of a UbL domain and at least one UBA domain and are thought to be able to shuttle proteins for degradation and function as proteasome substrate adaptors [2] , [24] . 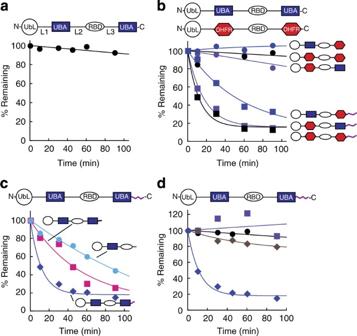Figure 1: Rad23 escapes proteasome degradationin vitrobecause it lacks an initiation region. The amount of protein remaining over time was plotted as a percentage of the initial total protein as described in the Methods section. (a) Degradation kinetics of Rad23. Incubation of Rad23 with purified yeast proteasome did not lead to its degradation at 30 °C. (b) The stability of Rad23 was not due to the UBA2 domain. Both UBA domains were replaced by dihydrofolate reductase (DHFR) individually or in combination and none of the substrates were degraded by the proteasome. Appending a 95 amino-acid unstructured region fromS. cerevisiaecytochromeb2to the C terminus of any of the Rad23 hybrid proteins in which either or both of the UBA domains had been replaced with a DHFR domain led to its rapid degradation. (c) Adding an initiation region to Rad23 led to its rapid degradation. Unstructured tails of different lengths were placed at the C terminus of Rad23 to serve as initiation regions. Rad23 with either a 39 amino-acid unstructured region from theE. colilac repressor (pink squares) or a 95 amino-acid unstructured region fromS. cerevisiaecytochromeb2(blue diamonds) added as an initiation region led to its degradation. Deletion of the UBA2, leaving a 45 amino-acid unstructured region, led to Rad23's degradation (light blue circles). (d) Degradation of Rad23 with a 95 amino-acid initiation region at its C terminus was proteasome dependent. Rad23-95 was stable when the proteasome was inhibited with MG132 (purple squares), in the absence of ATP (brown diamonds) in the degradation reaction, when its UbL domain was deleted (black circles). Rad23-95 was otherwise rapidly degraded by the proteasome (navy diamonds). Data points represent mean values and were calculated from at least three repeat experiments. Figure 1: Rad23 escapes proteasome degradation in vitro because it lacks an initiation region. The amount of protein remaining over time was plotted as a percentage of the initial total protein as described in the Methods section. ( a ) Degradation kinetics of Rad23. Incubation of Rad23 with purified yeast proteasome did not lead to its degradation at 30 °C. ( b ) The stability of Rad23 was not due to the UBA2 domain. Both UBA domains were replaced by dihydrofolate reductase (DHFR) individually or in combination and none of the substrates were degraded by the proteasome. Appending a 95 amino-acid unstructured region from S. cerevisiae cytochrome b 2 to the C terminus of any of the Rad23 hybrid proteins in which either or both of the UBA domains had been replaced with a DHFR domain led to its rapid degradation. ( c ) Adding an initiation region to Rad23 led to its rapid degradation. Unstructured tails of different lengths were placed at the C terminus of Rad23 to serve as initiation regions. Rad23 with either a 39 amino-acid unstructured region from the E. coli lac repressor (pink squares) or a 95 amino-acid unstructured region from S. cerevisiae cytochrome b 2 (blue diamonds) added as an initiation region led to its degradation. Deletion of the UBA2, leaving a 45 amino-acid unstructured region, led to Rad23's degradation (light blue circles). ( d ) Degradation of Rad23 with a 95 amino-acid initiation region at its C terminus was proteasome dependent. Rad23-95 was stable when the proteasome was inhibited with MG132 (purple squares), in the absence of ATP (brown diamonds) in the degradation reaction, when its UbL domain was deleted (black circles). Rad23-95 was otherwise rapidly degraded by the proteasome (navy diamonds). Data points represent mean values and were calculated from at least three repeat experiments. Full size image Surprisingly, Rad23 itself is not degraded despite its association with the proteasome [3] , [14] . Previous work has suggested that the second UBA domain of Rad23 (UBA2) is responsible for this stability [25] . The UBA2 domain can bind to Rad23's own UbL domain [25] , [26] , which in turn could limit Rad23's ability to bind to the proteasome [26] , [27] . The interaction of UbL and UBA domains in Rad23 may also lead to the formation of dimers or even larger structures, which could affect the degradation of Rad23 (refs 20 , 22 , 28 ). In this study, we propose a different and more general explanation for the stability of Rad23 and UbL–UBA adaptors. The degradation signal or degron in most proteasome substrates has two components: a proteasome-binding tag, typically a polyubiquitin chain, and an initiation region in which the proteasome engages its substrate and begins to degrade [29] , [30] , [31] . We propose that Rad23 remains stable because it has only one of the two required components of the degron: it contains the proteasome-binding tag, the UbL domain in this case, but lacks an effective initiation region. As a result, the proteasome is unable to engage the bound Rad23 effectively, and the protein remains stable despite the fact that it can bind to the proteasome. Rad23 can be rendered a substrate for the proteasome by introducing initiation regions into the protein, either by placing an unstructured tail at the end of Rad23, or by lengthening its internal flexible linkers. Experiments with both Rad23 and simplified model proteins show that internal regions flanked by folded domains must be much longer to support proteasome initiation than the unstructured tails at the ends of proteins. The requirement for longer internal initiation regions is consistent with a proteasomal receptor for the initiation region that is buried and accessible through a channel. Rad23 is stable because it lacks an initiation site Rad23 is not degraded by the proteasome [3] ( Fig. 1a and Supplementary Fig. S1 ) and earlier work suggests that the stability of Rad23 requires its carboxy (C)-terminal UBA domain (that is, the UBA2 domain) [25] . To test this hypothesis, we replaced both UBA domains in Rad23 individually and in combination with the unrelated small protein dihydrofolate reductase (DHFR) and tested whether the hybrid proteins are degraded by purified 26S yeast proteasome. Rad23 and the various Rad23–DHFR hybrid proteins remained stable in these assays, including constructs in which the UBA2 domain was replaced with DHFR ( Fig. 1b ). The degradation signal or degron in most proteasome substrates has two components: a proteasome-binding tag and an initiation region. Given that Rad23 is targeted to the proteasome through its UbL domain [3] , [14] , [15] , [16] , [18] we asked whether Rad23 lacked an initiation region. To address this question, we constructed Rad23 hybrids in which unstructured tails were attached to the C terminus of Rad23. The tails were derived either from the first 95 amino acids of the Saccharomyces cerevisiae cytochrome b 2 protein or from the 34 amino acids from an internal region of the Escherichia coli lac repressor (residues 321–354 of lacI) [32] , connected to Rad23 by a short linker. Both fusion proteins were degraded efficiently ( Fig. 1c and Supplementary Fig. S1 ). Deleting the UBA2 domain from Rad23 also creates an unstructured tail at the C terminus of the protein formed largely by linker residues that follow the RBD domain. This mutant Rad23 was also degraded, presumably because the newly exposed C-terminal tail could serve as an initiation region ( Fig. 1c ). Finally, addition of C-terminal tails also led to the degradation of the Rad23–DHFR hybrids discussed in the preceding paragraph ( Fig. 1b ). Three observations suggest that the Rad23 hybrids containing unstructured tails were degraded by the proteasome: degradation depended on the proteasome-binding UbL domain in the substrate ( Fig. 1d and Supplementary Fig. S1 ); degradation depended on the presence of ATP in the reaction mixture ( Fig. 1d ); and the proteasome inhibitor MG132 strongly inhibited degradation ( Fig. 1d ). Internal initiation sites in Rad23 are not very efficient The unstructured linker regions of Rad23 range in length from 45 to 82 amino acids. Sequences of similar lengths, 39 and 95 amino acids, derived from yeast cytochrome b 2 functioned as initiation sites when placed at the C terminus of Rad23 ( Fig. 1c ). Therefore, we asked why the linkers connecting the Rad23 domains did not serve as initiation regions for the proteasome. One possible explanation is that the amino acid sequence of the linkers itself was somehow responsible for the lack of degradation. To test this possibility, we replaced the linker regions with sequences of identical length also derived from the cytochrome b 2 . These hybrids were degraded faster than wild-type Rad23, but still only inefficiently ( Fig. 2a ). Thus, although the sequence identity of the linker region affected degradation, the length of the linker itself appears to impede the initiation of degradation. 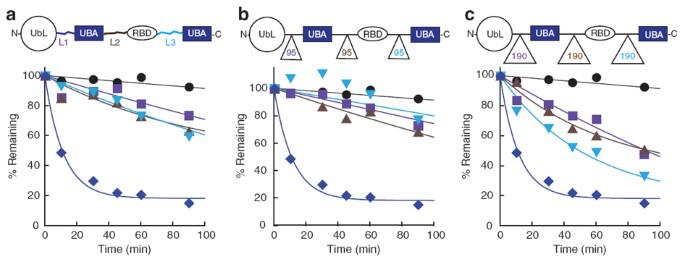Figure 2: Internal loops of Rad23 are too short to serve as effective initiation regions. Degradation kinetics at 30 °C are shown for Rad23 substrates with different linker regions. The amount of protein remaining over time was plotted as a percentage of the initial total protein as described in the Methods section. Degradation kinetics of Rad23 (black circles) and Rad23-95 (navy diamonds) are shown for comparison. (a) The amino acid sequences of the linker regions of Rad23 were not responsible for the lack of degradation. Replacement of linker regions L1 (purple squares), L2 (brown triangles), and L3 (light blue triangles) with a sequence fromS. cerevisiaecytochromeb2of the same length resulted in inefficient degradation by the proteasome. (b,c) Initiation regions have to be longer within a protein than at the end of a protein. Insertion of 95 (b) or 190 (c) amino-acid long sequences into linkers L1 (purple squares), L2 (brown triangles), and L3 (light blue triangles) led to increasing degradation of the hybrid proteins. Data points represent mean values and were calculated from at least three repeat experiments. Figure 2: Internal loops of Rad23 are too short to serve as effective initiation regions. Degradation kinetics at 30 °C are shown for Rad23 substrates with different linker regions. The amount of protein remaining over time was plotted as a percentage of the initial total protein as described in the Methods section. Degradation kinetics of Rad23 (black circles) and Rad23-95 (navy diamonds) are shown for comparison. ( a ) The amino acid sequences of the linker regions of Rad23 were not responsible for the lack of degradation. Replacement of linker regions L1 (purple squares), L2 (brown triangles), and L3 (light blue triangles) with a sequence from S. cerevisiae cytochrome b 2 of the same length resulted in inefficient degradation by the proteasome. ( b , c ) Initiation regions have to be longer within a protein than at the end of a protein. Insertion of 95 ( b ) or 190 ( c ) amino-acid long sequences into linkers L1 (purple squares), L2 (brown triangles), and L3 (light blue triangles) led to increasing degradation of the hybrid proteins. Data points represent mean values and were calculated from at least three repeat experiments. Full size image To test this hypothesis, we inserted 95 amino-acid long sequences that conferred instability to Rad23 when appended to the C terminus ( Fig. 1c ) into each of the three unstructured linker regions and followed the subsequent degradation by the proteasome ( Fig. 2b ). Surprisingly, these extended unstructured regions still did not function as efficient initiation sites ( Fig. 2b ). Only when we increased the length of the linkers even further by inserting a second 95 amino-acid long sequence into each of the linker regions were the constructs degraded by the proteasome ( Fig. 2c and Supplementary Fig. S1 ) with an efficiency approaching that of the C-terminal tails ( Fig. 1c ). These results suggested that the linker regions present in native Rad23 are not long enough to initiate degradation. Internal initiation requires long unstructured regions In Rad23, internal initiation regions needed to be considerably longer than initiation regions added as tails to function. Next, we asked whether this requirement is specific to Rad23 or characteristic of the length requirements for internal and terminal initiation in general. To address this question, we constructed a series of model proteins consisting of the UbL domain from Rad23 attached to the N terminus of a DHFR domain. We then added sequences derived from S. cerevisiae cytochrome b 2 either at the C terminus of the DHFR domain ( Fig. 3a ) or internally between the UbL and DHFR domains ( Fig. 3b and Supplementary Fig. S2 ). 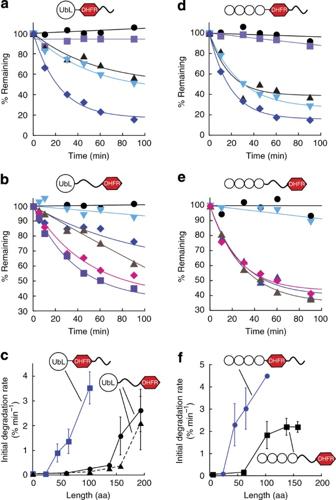Figure 3: Initiation length requirements for proteasomal degradation in model proteins. The model substrates with terminal initiation regions contained a UbL or Ub4domain attached to a DHFR domain followed by unstructured regions of different lengths at the C terminus. The substrates with internal initiation regions contained a UbL or Ub4domain attached to different length unstructured regions followed by a DHFR domain. Degradation experiments were performed at 30 °C. The amount of protein remaining over time was plotted as a percentage of the initial total protein as described in the Methods section. For all types of constructs degradation rates increased with the length of the initiation region. (a) Degradation reactions of UbL-containing substrates with C-terminal initiation regions. The tails consisted of 0 (black circles), 23 (purple squares), 44 (grey triangles), 64 (light blue triangles) and 102 (navy diamonds) amino acids derived fromS. cerevisiaecytochromeb2. (b) Degradation reactions of UbL-containing substrates with internal initiation regions, which consisted of 0 (black circles) 60 (light blue triangles), 102 (navy diamonds), 137 (brown triangles), 157 (pink diamonds) and 193 (purple squares) amino acids derived fromS. cerevisiaecytochromeb2. (c) Initial degradation rates were plotted against the length of the initiation region given as the number of amino acids (aa). Considerably longer initiation regions are required to support robust degradation when these regions are flanked by folded domains than when they are placed at the C terminus of the substrates. The requirement for long initiation regions does not appear to depend on the details of the amino acid sequence of the initiation region as scrambling the amino acid sequence of the linkers used (black dotted line) did not change the initiation region length dependence of degradation significantly. (d) Degradation reactions of ubiquitin-tagged substrates with C-terminal initiation regions; initiation regions were the same as ina. (e) Degradation reactions of ubiquitin-tagged substrates with internal initiation regions; initiation regions are the same as inb. (f) Initial degradation rates of ubiquitin-tagged substrates plotted against the length of the initiation region given as the number of amino acids. Data points represent mean values and error bars show standard errors calculated from at least three repeat experiments. Figure 3: Initiation length requirements for proteasomal degradation in model proteins. The model substrates with terminal initiation regions contained a UbL or Ub 4 domain attached to a DHFR domain followed by unstructured regions of different lengths at the C terminus. The substrates with internal initiation regions contained a UbL or Ub 4 domain attached to different length unstructured regions followed by a DHFR domain. Degradation experiments were performed at 30 °C. The amount of protein remaining over time was plotted as a percentage of the initial total protein as described in the Methods section. For all types of constructs degradation rates increased with the length of the initiation region. ( a ) Degradation reactions of UbL-containing substrates with C-terminal initiation regions. The tails consisted of 0 (black circles), 23 (purple squares), 44 (grey triangles), 64 (light blue triangles) and 102 (navy diamonds) amino acids derived from S. cerevisiae cytochrome b 2 . ( b ) Degradation reactions of UbL-containing substrates with internal initiation regions, which consisted of 0 (black circles) 60 (light blue triangles), 102 (navy diamonds), 137 (brown triangles), 157 (pink diamonds) and 193 (purple squares) amino acids derived from S. cerevisiae cytochrome b 2 . ( c ) Initial degradation rates were plotted against the length of the initiation region given as the number of amino acids (aa). Considerably longer initiation regions are required to support robust degradation when these regions are flanked by folded domains than when they are placed at the C terminus of the substrates. The requirement for long initiation regions does not appear to depend on the details of the amino acid sequence of the initiation region as scrambling the amino acid sequence of the linkers used (black dotted line) did not change the initiation region length dependence of degradation significantly. ( d ) Degradation reactions of ubiquitin-tagged substrates with C-terminal initiation regions; initiation regions were the same as in a . ( e ) Degradation reactions of ubiquitin-tagged substrates with internal initiation regions; initiation regions are the same as in b . ( f ) Initial degradation rates of ubiquitin-tagged substrates plotted against the length of the initiation region given as the number of amino acids. Data points represent mean values and error bars show standard errors calculated from at least three repeat experiments. Full size image The proteasome did not degrade substrates with 23 amino-acid long tails, but degradation rates increased progressively and substantially as the tails were extended to 44, 64 and 102 amino acids ( Fig. 3a,c ), in accord with earlier studies [30] , [33] . This effect was not a result of the specific amino acid sequences of the tails added, as scrambling the amino acid sequences of the tails yielded equivalent results ( Fig. 3c ). When sequences were inserted between the folded UbL and DHFR domains, degradation rates increased only slowly as a function of length ( Fig. 3b,c ) compared with constructs with the same sequences appended at the C terminus ( Fig. 3a,c ). For example, a 60 amino acid tail at the end of a UbL–DHFR fusion allowed the protein to be degraded rapidly, but the same 60 amino acids inserted between the UbL and DHFR domains did not allow this protein to be degraded. An insert had to be at least 137 amino acids for slow degradation to occur and 157 amino acids or more for rapid degradation ( Fig. 3b,c ). The inserted linkers are unstructured because they are highly sensitive to added nonspecific proteases, whereas the DHFR domain resisted proteolysis ( Supplementary Fig. S3 ); inserting a linker of similar length but containing a folded domain did not allow degradation ( Supplementary Fig. S4 ). In addition, the DHFR domain is stabilized by the ligand methotrexate, again suggesting that it is in its native conformation ( Supplementary Fig. S3 ). One explanation of these results could be that the longer initiation regions led to degradation because the longer inserts introduced amino acid sequences that contained a proteasome recognition motif. However, two observations suggest that the actual length of the inserts is responsible for degradation. First, the inserts longer than 95 amino acids in length were constructed as partial repeats of the first 95 amino acids ( Supplementary Fig. S2 ), therefore the longer inserts do not contain new amino acid sequences. Second, repeating the experiments with linkers derived from a scrambled amino acid sequence ( Fig. 3c ) or an unrelated sequence derived from subunit 9 of the F o ATPase ( Supplementary Fig. S5 ) yielded similar results. Therefore, we concluded that the behaviour of Rad23 reflects a general mechanism, namely that degradation from internal regions requires much longer initiation regions than degradation from tails at the end of proteins. Targeting tags affect initiation region length requirements UbL domains are found in proteins associated with the proteasome, but most proteins seem to be targeted for proteasome degradation by ubiquitin modifications. To determine whether the requirements for initiation regions were specific to the UbL domain, we tested whether proteasome substrates targeted by ubiquitin tags also required long internal initiation regions for rapid degradation. To do so, we constructed proteins that contained the same DHFR domain and initiation regions as before, but the UbL domain was replaced with four ubiquitin moieties fused in frame N to C termini [34] , [35] . This linear ubiquitin tag is known to target proteins to the proteasome for degradation both in vitro and in vivo [34] . The substrates with the ubiquitin tag no longer contained any components derived from Rad23 but also required long internal initiation regions to be degraded ( Fig. 3d–f ). These internal initiation regions again needed to be much longer than when they were added as tails ( Fig. 3f ). Interestingly, internal loops could be somewhat shorter with ubiquitin tags than with UbL tags and still serve as effective initiation regions ( Fig. 3c,f ). However, the main conclusion of this set of experiments is that the requirement for the much greater length of unstructured regions serving as internal initiation sites compared with terminal initiation sites reflects a general property of the proteasome; it is independent of the origin of the substrate protein or the proteasome-binding tag. Initiation sites determine Rad23 stability in vivo The experiments described above demonstrate that Rad23 stability can be controlled through the addition of a proteasome initiation site in a well-defined, in vitro reconstituted proteasome degradation system. In vivo , the stability of Rad23 may be affected by additional factors such as non-stoichiometric proteasome subunits lost during purification, components of the ubiquitination machinery or Rad23-binding partners. To test whether the stability of Rad23 in vivo was also due to the absence of an initiation site, we measured the accumulation of Rad23 hybrid proteins in yeast. To follow the expression of Rad23 hybrids in the background of wild-type Rad23, we expressed constructs containing an N-terminal Flag tag in S. cerevisiae under the control of a strong constitutive promoter. The Flag tag did not destabilize Rad23 and tagged Rad23 accumulated in yeast. The host strain was deleted for the PDR5 gene, which encodes a plasma membrane ATP-binding cassette transporter. Deleting this transporter renders the yeast more sensitive to drugs, including proteasome inhibitors (for example, see ref. 36 ). The Rad23 hybrid proteins accumulated to different levels when expressed in yeast. Appending 39 or 95 amino-acid long tails at the C terminus of Rad23 (to create Rad23-39 and Rad23-95) resulted in the disappearance of detectable levels of the hybrid protein ( Fig. 4 ). The genes for these constructs were expressed at levels at least equal to those of the RAD23 gene lacking a tail, demonstrating that the observed decreases in protein levels were caused by post-transcriptional regulation ( Supplementary Fig. S6 ). Indeed, Rad23-39 and Rad23-95 accumulated when the proteasome was inhibited with MG132 ( Fig. 4 ). In vitro , the 95 amino-acid tail led to more rapid degradation than shorter tails ( Fig. 1c ) and correspondingly less Rad23-95 than Rad23-39 accumulated in vivo ( Fig. 4 ), presumably because not all proteasome activity was inhibited by the addition of MG132. Rad23-95 accumulated when its UbL domain was deleted (data not shown). Rad23 remains stable when its UBA domains are replaced with DHFR domains ( Supplementary Fig. S7 ). This observation suggests that the stabilizing effect of these domains is due to a general property of compact structures. 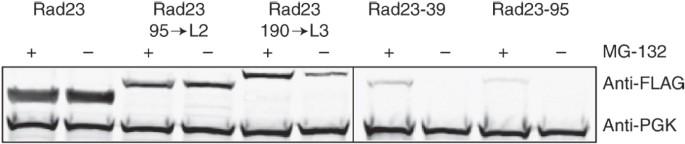Figure 4: The stability of Rad23in vivois also determined by the presence of an initiation region. Rad23 with an N-terminal Flag tag expressed inS. cerevisiaeaccumulated and protein levels were not affected by MG132 as determined by western blotting for the Flag tag in yeast extracts. Addition of a 39 amino-acids long tail to the C terminus of Rad23 (Rad23-39) or insertion of a 190 amino-acid long linker into loop 3 (Rad23-190L3) destabilized the protein and reduced steady-state levels in the cell. Inhibition of proteasomal degradation with MG132 stabilized the Rad23 variants and increased their steady-state levels. Rad23 with a 95 amino-acid long tail (Rad23-95) was barely detectable even when the proteasome was inhibited with MG132, but deletion of the UbL domain stabilized the protein sufficiently to allow it to accumulate (not shown). Insertion of a 95 amino-acid linker into loop 2 did not destabilize the protein noticeably (Rad23-95L2). No Flag-tagged Rad23 was detected in lysate of cells transformed with plasmid lacking the Rad23 insert (data not shown) and phosphoglycerate kinase (PGK) was measured as a loading control to allow comparison of protein levels in the different lysates. Figure 4: The stability of Rad23 in vivo is also determined by the presence of an initiation region. Rad23 with an N-terminal Flag tag expressed in S. cerevisiae accumulated and protein levels were not affected by MG132 as determined by western blotting for the Flag tag in yeast extracts. Addition of a 39 amino-acids long tail to the C terminus of Rad23 (Rad23-39) or insertion of a 190 amino-acid long linker into loop 3 (Rad23-190 L3) destabilized the protein and reduced steady-state levels in the cell. Inhibition of proteasomal degradation with MG132 stabilized the Rad23 variants and increased their steady-state levels. Rad23 with a 95 amino-acid long tail (Rad23-95) was barely detectable even when the proteasome was inhibited with MG132, but deletion of the UbL domain stabilized the protein sufficiently to allow it to accumulate (not shown). Insertion of a 95 amino-acid linker into loop 2 did not destabilize the protein noticeably (Rad23-95 L2). No Flag-tagged Rad23 was detected in lysate of cells transformed with plasmid lacking the Rad23 insert (data not shown) and phosphoglycerate kinase (PGK) was measured as a loading control to allow comparison of protein levels in the different lysates. Full size image Internal initiation sites also functioned in vivo. Inserting a 190 amino-acid loop into the L3 region of Rad23 significantly reduced the amount of the hybrid protein relative to that of the wild-type Rad23 ( Fig. 4 ). Proteasome degradation apparently caused the destabilization, as protein levels were restored by its inhibitor MG132 ( Fig. 4 ). Degradation in vivo appears to follow the same length requirements as degradation in vitro ; inserting a 95 amino-acid loop into the L2 region of Rad23 had little effect on protein levels relative to wild-type Rad23 ( Fig. 4 ), just as observed in vitro ( Fig. 2b ). In summary, the stability of hybrid Rad23 proteins in vivo behaved as predicted from the in vitro proteasome degradation assays. Thus, it appears that also in vivo Rad23 escapes proteasome degradation because it lacks an effective initiation region. Initiation is governed by the same length requirements for initiation in vivo as in vitro . Rad23 binds the proteasome and ubiquitinated proteins, which are subsequently degraded, but Rad23 itself escapes to shuttle the next round of substrates for degradation. The fact that Rad23 escapes proteolysis makes it a more effective and efficient proteasome adaptor. Understanding the molecular mechanism by which Rad23 avoids proteolysis should provide clues regarding the selection of substrates by the proteasome. Here, we propose that Rad23 lacks a critical part of the degron, the proteasome initiation region. This hypothesis is supported by the observation that introducing unstructured linkers into various regions of Rad23 to serve as artificial initiation regions led to Rad23's rapid proteolysis both in vitro ( Figs 1 and 2 ) and in vivo ( Fig. 4 ). Previous studies that investigated the stability of Rad23 strongly implicated a specific function of the C-terminal UBA2 domain of Rad23 in its stabilization [25] . However, the experimental findings on which this conclusion was based may also fit the simpler model described here. Destabilizing the UBA2 domain with a single amino acid substitution or deleting it entirely leads to the rapid degradation of Rad23 (ref. 25 ). The proteins Ddi1 and Dsk2 (ref. 25 ; see below) as well as human protein ataxin-1 interacting ubiquitin-like protein [37] also contain N-terminal UbL domains and C-terminal UBA domains. Just like Rad23, these proteins accumulate in the cytosol but become rapidly degraded when their UBA domains are mutated [25] , [37] . However, at least for Rad23, it appears to be simply the compact structure of the UBA2 domain that is important for Rad23 stability and replacing the UBA2 domain with a DHFR domain did not destabilize Rad23 ( Fig. 1b ). The amino acid sequences of the UBA2 domain and DHFR are not related to each other and therefore the proteins are not expected to interact with the same partners. The mutations in the UBA2 domain destabilized the structure [25] and it is possible that they did so sufficiently so that it unfolded and served as an unstructured initiation region. Similarly, deleting the UBA2 domain leaves a 45 amino-acid tail at the C terminus of Rad23 that in turn can serve as the proteasome initiation region ( Fig. 1c ). This mechanism is also consistent with the finding that deleting the last ten amino acids of the UBA2 domain leads to Rad23's rapid degradation [3] . Protein folding is highly cooperative so that deleting even a small number of amino acids from a folded domain leads to its unfolding (for example, see ref. 38 ). Finally, it has been observed that attaching an epitope tag to the C terminus of Rad23 can lead to its rapid degradation by the proteasome in vivo [3] , presumably because the tag provides a proteasome initiation site. The structured domains in Rad23 are connected by relatively long loops that are flexible in the human Rad23 homologue HR23a [13] . The proteasome does not initiate degradation at these loops, despite the fact that extensions of similar lengths attached to the end of Rad23 lead to its rapid degradation ( Figs 1c and 4 ). Indeed, experiments with model proteins suggest that internal loops flanked by folded domains must be surprisingly long and in the range of 150 amino acids or more to support rapid degradation ( Fig. 3 ). Interestingly, it seems that the upper lengths of linkers found in Rad23 homologues are always below this 150 amino acid cutoff ( Fig. 5 ). A comparison of the amino acid sequences of fifteen Rad23 proteins from a broad range of eukaryotes ( Fig. 5 and Supplementary Information ) suggests that the sequences of the folded domains in these homologues (that is, the UbL, UBA and RBD domains) are well conserved but that the sequences of the linkers connecting the domains are much less so ( Fig. 5b ). The linker lengths vary considerably, ranging from 13 to 114 amino acids, but the lengths of the linkers always stays below the length that would be required for proteasomal degradation ( Fig. 5c ). 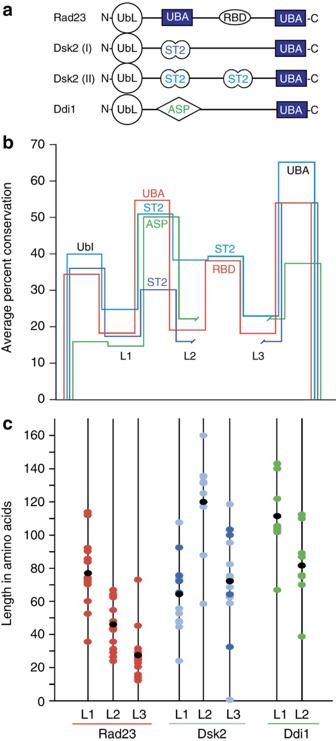Figure 5: Analysis of loops within UbL–UBA proteins. Homologues of Rad23, Dsk2 and Ddi1 were retrieved from species selected broadly from evolution (seeSupplementary Information). The loops within these proteins are defined as sequences that fall between motifs found in the SMART59and Pfam41databases. (a) Schematic of UbL–UBA proteins. Domains and loops represented are not to scale. In addition to UbL and UBA, abbreviations include ST2 (Sti1/Sti1 pair) and ASP (Asp_protease). Note that Rad4-binding domain (RBD) corresponds to the Pfam domain XPC. (b) Relative conservation of domains and loops. Conservation was evaluated by aligning individual domains with Clustal W60, extracting the pairwise percent conservation and averaging. Domains are represented by horizontal segments. Rad23 is shown in red, Dsk2 class I and II are shown in dark and light blue, respectively, and Ddi1 is shown in green. To align all of the UBA domains in the schematic, break points are introduced into the traces for class I Dsk2 and Ddi1. (c) Plot of loop lengths. The colour scheme for the loops is continued fromb. Black dots indicate the average loop length. Figure 5: Analysis of loops within UbL–UBA proteins. Homologues of Rad23, Dsk2 and Ddi1 were retrieved from species selected broadly from evolution (see Supplementary Information ). The loops within these proteins are defined as sequences that fall between motifs found in the SMART [59] and Pfam [41] databases. ( a ) Schematic of UbL–UBA proteins. Domains and loops represented are not to scale. In addition to UbL and UBA, abbreviations include ST2 (Sti1/Sti1 pair) and ASP (Asp_protease). Note that Rad4-binding domain (RBD) corresponds to the Pfam domain XPC. ( b ) Relative conservation of domains and loops. Conservation was evaluated by aligning individual domains with Clustal W [60] , extracting the pairwise percent conservation and averaging. Domains are represented by horizontal segments. Rad23 is shown in red, Dsk2 class I and II are shown in dark and light blue, respectively, and Ddi1 is shown in green. To align all of the UBA domains in the schematic, break points are introduced into the traces for class I Dsk2 and Ddi1. ( c ) Plot of loop lengths. The colour scheme for the loops is continued from b . Black dots indicate the average loop length. Full size image The proposed mechanism explaining the stability of Rad23 could apply to the behaviour of other cellular proteins. For example, Rad23 is a member of a larger group referred to as UbL/UBA proteins because they all contain at least one domain of this kind. Other members of this group in yeast, Ddi1 and Dsk2, are structurally and functionally similar to Rad23 and, as mentioned above, they each contain an N-terminal UbL domain but only one C-terminal UBA domain [2] , [24] . Both proteins bind to the proteasome by their UbL domains and to ubiquitinated proteins through their C-terminal UBA domain. Thus, like Rad23, Ddi1 and Dsk2 function as ubiquitin receptors and facilitate transport of ubiquitinated proteins to the proteasome for degradation [2] , [19] , [21] , [23] , [24] . Ddi1, for example, is responsible for the proteasomal degradation of Ho endonuclease and the deletion of Ddi1 results in the stabilization of Ho protein in vivo [39] . Dsk2 has a role in the UFD proteolytic pathway [21] , [40] and in the proteasomal degradation of N-end rule model substrates by binding to K48-linked polyubiquitin chains [23] . Interestingly, and similarly to Rad23, there is no evidence of proteasomal degradation of either Ddi1 or Dsk2, regardless of their association with the proteasome [3] , [14] , [25] . Comparing the sequences of twenty four Ddi1 and Dsk2 homologues from a range of eukaryotic species shows again that the folded domains in these proteins are more conserved than the loops ( Fig. 5b ). The lengths of the loops vary as they did for Rad23 but the upper limit again coincides with the cutoff for internal proteasome initiation sites and the requirement of these proteins to avoid degradation ( Fig. 5b ). The loops connecting domains in Rad23 have unusual amino acid compositions, and large fractions of these loops have been annotated as low complexity regions in the PFAM database [41] , meaning that one or a few amino acids are overrepresented. In principle, this amino acid composition could also affect how well the loops serve as proteasome initiation sites. Indeed, we found that stretches of a strongly biased amino acid composition adjacent to a folded domain can block proteasome progression and may allow some substrates to escape from the proteasome before they are fully degraded [42] , [43] . The amino acid composition of the Rad23 loops is not responsible for the stability of the protein because replacing the loops with peptides of different and unbiased sequences does not substantially destabilize Rad23. However, this finding does not rule out that amino acid composition has an effect on the ability of peptides to serve as initiation sites. Indeed, the Rad23 loops do not function well as initiation sites when tested in model proteasome substrates ( Supplementary Fig. S8 ), and any effects of amino acid composition on proteasome initiation will need to be investigated in the future. The long length requirement for internal proteasome initiation sites probably has a structural explanation. If, as seems likely (see below), the receptor for initiation regions is located in a channel in the proteasome, folded domains would block access to the binding site. Depending on how deeply the receptor is buried, long flexible linkers would be required to reach the binding site. In the simplest case, twice the length of linkers would be required when folded domains block both ends of the initiation region than when one end is open ( Fig. 6 ). However, other geometries are also possible and could lead to similar results. The location of the initiation site receptor on the proteasome is unknown, but the bacterial degradation system provides some clues. In bacteria, the functions of the proteasome are performed by AAA+ proteases, which share their architecture with the proteasome and appear to work by the same overall mechanism [44] , [45] . Proteins are targeted to AAA+ proteases by linear peptide sequences that perform the same function as the degradation initiation sites in proteasome substrates (for example, refs 46 , 47 , 48 ). The AAA+ proteases recognize these targeting signals with loops that are lining the degradation channel [49] , [50] , [51] , [52] . Because of the similarities between the proteasome and the AAA+ proteases, the proteasome may recognize initiation sites in the same way. The proteasome degradation channel is narrow but it can accommodate two polypeptide chains simultaneously [53] , and therefore should allow the insertion of a polypeptide loop during the initiation of degradation. 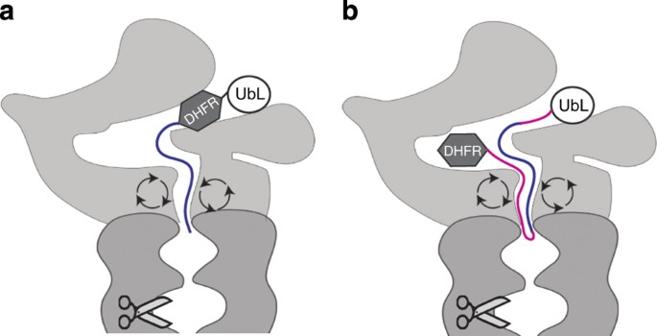Figure 6: Schematic representation of the length requirement for internal and terminal initiation regions. Substrates shown contained a UbL domain bound to the proteasome in an arbitrary position attached to either a dihydrofolate reductase (DHFR) domain followed by an initiation region (blue) or an initiation region (red and blue) followed by a DHFR domain. Length requirements for an internal initiation region (red and blue) were at least twice that for a terminal initiation region (blue). Light grey, proteasome caps; dark grey, proteasome core; circular arrows, ATPase subunits; scissors, proteolytic sites. Figure 6: Schematic representation of the length requirement for internal and terminal initiation regions. Substrates shown contained a UbL domain bound to the proteasome in an arbitrary position attached to either a dihydrofolate reductase (DHFR) domain followed by an initiation region (blue) or an initiation region (red and blue) followed by a DHFR domain. Length requirements for an internal initiation region (red and blue) were at least twice that for a terminal initiation region (blue). Light grey, proteasome caps; dark grey, proteasome core; circular arrows, ATPase subunits; scissors, proteolytic sites. Full size image Substrates that were targeted to the proteasome by a ubiquitin tag instead of a UbL tag appeared to need somewhat shorter internal initiation regions for effective degradation. In the model proposed above, the simplest explanation for this observation would be that the UbL receptor on the proteasome is located further from the initiation region receptor than the ubiquitin receptors, as has been suggested recently from protein degradation experiments [54] . An alternative explanation for the inefficient initiation from internal sites could be that the proteasome is simply not able to unfold two domains at the same time. The proteasome unravels structured domains in a substrate sequentially after it begins degradation at one of the ends of the polypeptide chain [44] and it can do so very effectively [55] . When the proteasome initiates between two domains, it may fail at this task if forced to unfold them both at the same time [56] . However, the observation that simply lengthening internal initiation regions allows degradation to occur suggests that the proteasome is able to cope with two domain substrates, either by unravelling these domains sequentially or simultaneously. Where the proteasome fails to degrade one or both domains, the most likely outcome is clipping of the substrate rather than failure to initiation [56] . In summary, we propose that Rad23 escapes proteasome degradation because it lacks a critical part of the degron, namely an initiation region. Unstructured regions in proteins often initiate degradation, but the unstructured regions in Rad23 are flanked by folded domains and probably cannot reach the initiation receptor of the proteasome. Degradation from an internal site requires long unstructured initiation regions. Creating initiation sites in Rad23 by lengthening its internal linkers leads to the protein's rapid proteasomal degradation. We propose that the requirement for long internal initiation regions for proteasome degradation also explains the stability of other proteins in the cell, such as the UbL/UBA family of adaptor proteins. Substrate proteins Protein substrates were derived from S. cerevisiae Rad23 and E. coli DHFR; the unstructured regions were derived from either residues 1–95 of S. cerevisiae cytochrome b 2 or residues 321–354 of the E. coli lac repressor [32] . Lysines in these sequences were replaced by arginines unless noted otherwise. For in vitro experiments, constructs were cloned into the plasmid pGEM-3Zf (+) (Promega), where they were under the control of the T7 promoter; for in vivo experiments, constructs were cloned into the yeast CEN vector p416 GPD in which they were under the control of the strong, constitutive glyceraldehyde-3-phosphate dehydrogenase (GPD) promoter [57] . One set of model protein constructs contained the UbL domain and the following 22 residues of S. cerevisiae Rad23 (that is, amino acid 1–99 of Rad23) as well as E. coli DHFR. Unstructured regions consisting of different combinations of residues 1–95 of cytochrome b 2 were inserted between UbL and DHFR with short linkers. Specifically, the construct UbL-60-DHFR consisted of amino acids 1–55 of cytochrome b 2 , the construct UbL-102-DHFR consisted of amino acids 1–95, UbL-137-DHFR consisted of amino acids 1–95 followed by amino acids 1–35, UbL-157-DHFR consisted of amino acids 1–95 followed by amino acids 1–55 and UbL-193-DHFR consisted of two repeats of amino acids 1–57 of cytochrome b 2 followed by amino acids 1–55 of cytochrome b 2 . In the constructs with the unstructured regions on the C terminus of DHFR, different parts of the cytochrome b 2 sequence were followed by a hexahistidine tag. Specifically, the constructs UbL-DHFR-23, UbL-DHFR-44 and UbL-DHFR-64 consisted of the first 8, 28 and 48 amino acids, respectively, each followed by amino acids 90–95. UbL-DHFR-102 consisted of amino acids 1–95. The scrambled initiation regions were derived from the first 51 amino acids of S. cerevisiae cytochrome b 2 and the sequence QRTLSRSFYSTATGAASRSGR (derived from cytochrome c 1 ). This sequence was then scrambled using a scrambling algorithm. The resulting sequence was optimized for E. coli codon usage and common restriction sites were removed with the web-based sequence tool DNAWorks ( http://mcl1.ncifcrf.gov/dnaworks ) and the gene was constructed by PCR assembly. In the ubiquitin-tag constructs, the coding region for the UbL domain and the following 22 residues of S. cerevisiae Rad23 were replaced with four copies of the coding region for ubiquitin, each of which contains the mutation Gly 76 to Val, connecting each domain with the linker GSGGGG as described previously [34] . In the Rad23 constructs, sequences either replaced Rad23's linker regions, were inserted into the linker regions, or were attached to the C terminus of Rad23. The insertions in one set of Rad23 constructs consisted of amino acids 1–95 of cytochrome b 2 inserted after amino acid 111 of Rad23 to yield Rad23-95 L1, after amino acid 219 of Rad23 to yield Rad23-95 L2 and after amino acid 325 of Rad23 to yield Rad23-95 L3 constructs. In a second set of constructs, two repeats of amino acids 1–95 of cytochrome b 2 were inserted at the same positions to yield Rad23-190 L1, Rad23-190 L2 or Rad23-190 L3. Constructs with replacement sequences in the linker regions of Rad23, Rad23 ΔL1, Rad23 ΔL2 and Rad23 ΔL3, consisted of amino acids 1–71, 1–83 and 1–44, respectively, of cytochrome b 2 . The C-terminal tail construct Rad23-95 contained amino acids 1–95 of cytochrome b 2 attached to the C terminus of Rad23 and Rad23-39 contained amino acids 321–354 of the lac repressor attached to the C terminus of Rad23. All genes were constructed using standard molecular biology techniques and verified by DNA sequencing. Protein expression and purification Yeast proteasome was purified from S. cerevisiae strain YYS40 ( MATa rpn11 ∷ RPN11 3XFLAG -HIS3 leu2 his3 trp1 ade2 can1 ssd1 ). In this strain, the genomic copy of RPN11 is replaced with an RPN11 gene containing the coding sequence for three Flag tags at its 3′-end [58] . The 26S proteasome was purified using immunoaffinity chromatography using FLAG antibodies (M2-agarose affinity beads; Sigma) following the published protocol [58] with minor modifications. For in vitro degradation experiments, UbL-tagged radioactive substrates were expressed from a T7 promoter by in vitro transcription and translation using a TNT Coupled Reticulocyte Lysate System (Promega) containing [ 35 S] methionine. Ubiquitin-tagged radioactive substrates were expressed from a T7 promoter by in vitro transcription and translation using an E. coli T7 S30 Extract System for Circular DNA (Promega) containing [ 35 S] methionine. After synthesis, the substrates were partially purified by high-speed centrifugation followed by precipitation in two volumes of saturated ammonium sulphate. Substrates were incubated on ice for a minimum of 1 h, pelleted and resuspended in degradation buffer (5% [v/v] glycerol, 5 mM MgCl 2 , 50 mM Tris-HCl [pH 7.4]). Proteasome degradation assays Degradation assays were performed with 50 nM purified yeast proteasome, at 30 °C in 5% [v/v] glycerol, 5 mM MgCl 2 , 50 mM Tris-HCl (pH 7.4), 1 mM DTT and in the presence of an ATP-regeneration system (1 mM ATP, 10 mM creatine phosphate, 0.1 mg ml −1 creatine phosphokinase). In vitro -translated [ 35 S]-methionine-labelled proteins were added to purified proteasomes in reaction buffers to start degradation. Samples were withdrawn at the indicated times, added to SDS polyacrylamide gel electrophoresis (PAGE) sample buffers to stop the reactions and analysed by SDS–PAGE. The amounts of radioactive proteins were determined by electronic autoradiography (Instant Imager; Packard). Degradation experiments were each conducted at least three times and protein amounts plotted against degradation times. These data were fitted to equations describing single exponential decays, and initial degradation rates were calculated from the fit amplitudes and first-order rate constants. When the changes in protein amounts over the total reaction times were small, data were fit to straight lines as approximations of the initial phases of exponential decays and the slopes of lines taken as initial degradation rates. Curve fittings were performed with the graphing software package Kaleidagraph (version 4.0, Synergy Software). The error bars for initial degradation rates are standard errors obtained from at least three independent measurements. In vivo protein levels Rad23 fusion proteins were expressed under the control of the strong constitutive GPD promoter from a CEN plasmid (p416 GPD), with a URA3 marker gene [57] . These Flag-tagged constructs were used to transform S. cerevisiae strain BY4741pdr5 ( MATa his3Δ1 leu2Δ0 met15Δ0 ura3Δ0 pdr5 ∷ kanMX4 ) using standard protocols. Transformants were cultured overnight in an SC-Ura liquid medium at 30 °C, diluted to an OD 600 nm of 0.2, grown to a mid-log phase in the presence or absence of 200 μM MG132 and then collected by centrifugation. Cell pellets were suspended in a HEPES lysis buffer (8 M urea, 50 mM HEPES [pH7.4], 2.5% SDS) and lysed using glass beads (BioSpec Products) and vortexing. Proteins were separated by SDS–PAGE, transferred to a nitrocellulose membrane (Pall Corporation) and detected with a monoclonal anti-Flag antibody (Sigma) and an Alexa-800-labelled goat anti-mouse secondary antibody (Rockland Immunochemicals). Protein levels were quantified using an Odyssey infrared imaging system (Li-COR Biosciences) and normalized using phosphoglycerate kinase levels detected by an anti-PGK monoclonal antibody (Invitrogen) and an Alexa-800 goat anti-mouse secondary antibody (Rockland Immunochemicals). Transcription levels To measure the relative levels of mRNA expression for each Rad23 construct, we extracted RNA from yeast cultures containing the different Rad23 constructs using the RNeasy Mini Kit (Qiagen). Approximately 2 μg of total RNA was reverse transcribed using 6.3 μM oligo dT and reverse transcriptase at 42 °C for 1 h. Total product (50–100 ng) was used as the template for the quantitative PCR reactions using sets of primers specific to Flag-tagged Rad23 to distinguish transgene transcripts from those resulting from endogenous Rad23 expression. A primer set specific to actin was used as an internal control. The sequences of the primers used were the following: ACT1CDSF, 5′-GGTTATTGATAACGGTTCTGGTATG-3′; ACT1CDSR, 5′-ATGATACCTTGGTGTCTTGGTCTAC-3′; FLAG-Rad23F, 5′-GGGCGATTATAAAGATGATGACG-3′; FLAG-RAD23R, 5′-TGTGTTTGAAGGTTCCAGATC-3′. Serial dilutions of total yeast DNA and linear regression analysis of cycle threshold (Ct) values were used to establish standard curves of each primer set. Relative expression levels of each Rad23 transgene were determined using the standard curves for each primer set and normalized by dividing each sample value by actin expression levels. All reactions were carried out in triplicate. How to cite this article: Fishbain, S. et al . Rad23 escapes degradation because it lacks a proteasome initiation region. Nat. Commun. 2:192 doi: 10.1038/ncomms1194 (2011).